DPP6 regulation of dendritic morphogenesis impacts hippocampal synaptic development Dipeptidyl-peptidase 6 is an auxiliary subunit of Kv4-mediated A-type K + channels that, in addition to enhancing channel surface expression, potently accelerates their kinetics. The dipeptidyl-peptidase 6 gene has been associated with a number of human central nervous system disorders including autism spectrum disorders and schizophrenia. Here we employ knockdown and genetic deletion of dipeptidyl-peptidase 6 to reveal its importance for the formation and stability of dendritic filopodia during early neuronal development. We find that the hippocampal neurons lacking dipeptidyl-peptidase 6 show a sparser dendritic branching pattern along with fewer spines throughout development and into adulthood. In electrophysiological and imaging experiments, we show that these deficits lead to fewer functional synapses and occur independently of the potassium channel subunit Kv4.2. We report that dipeptidyl-peptidase 6 interacts with a filopodia-associated myosin as well as with fibronectin in the extracellular matrix. dipeptidyl-peptidase 6 therefore has an unexpected but important role in cell adhesion and motility, impacting the hippocampal synaptic development and function. A-type voltage-gated K + currents in the hippocampal CA1 pyramidal neurons act to dampen action potential initiation and frequency. Due to their high expression and hyperpolarized voltage for activation in dendrites, they control action potential back propagation into dendrites, contributing to synaptic integration and plasticity [1] . Somatodendritic A-type K + channels in the CA1 hippocampal pyramidal neurons are primarily composed of pore-forming Kv4.2 subunits [2] , [3] , which undergo activity-dependent trafficking in the hippocampal neurons [4] . Reconstitution of native A-current properties in heterologous systems appears to require the co-expression of Kv4.2 along with two auxiliary subunits: the Kv channel-interacting proteins and dipeptidyl aminopeptidase-like proteins [5] , [6] . Immunohistochemical staining studies suggest that CA1 pyramidal neurons primarily express KChIP2, KChIP4 and dipeptidyl-peptidase 6 (DPP6) proteins [7] , [8] . Recently genomewide-association studies have implicated DPP6 in autism spectrum disorders and other neuropsychiatric pathologies [9] , [10] . DPP6 interacts with Kv4 channels to dramatically increase Kv4 surface expression and accelerate many properties of A-type channels including their activation, inactivation and recovery from inactivation [11] , [12] . Recently, we found DPP6 to be particularly important for the localization of Kv4 channels to the distal CA1 dendrites [13] . Structurally, the DPP6 protein has a single transmembrane domain with a short intracellular amino terminus. The vast majority of the protein, however, consists of a large extracellular carboxy terminal domain [14] , [15] . The extracellular domain of a related family member, DPPIV (also termed CD26), binds to components of the extracellular matrix (ECM), like collagen, fibronectin and integrin β1 (refs 16 , 17 ) and mediates roles in cell adhesion, cellular trafficking and T-cell activation [18] , [19] , [20] . DPP6 has approximately 50% similarity to CD26 (ref. 21 ), and also has a cysteine-rich domain that may bind to components of the ECM. The function of DPP6’s extracellular domain is unknown but based on its prominence and similarity to that of DPPIV, it seemed possible that DPP6 may have a role in cell adhesion, subcellular recognition and/or trans-synaptic signalling. Here we show that the initiation and stability of dendritic filopodia are greatly reduced in DPP6 knockout (DPP6-KO) mouse hippocampal neurons. Moreover, dendritic tree size, spine density and functional synapse numbers are reduced throughout development and in adulthood in these mice. These deficiencies are rescued by expression of DPP6. While a profusion of recent research has greatly added to our comprehension of the molecules involved in the formation, maintenance and remodelling of spines, relatively little is known about the molecular and cellular mechanisms underlying the formation and maintenance of dendritic filopodia. Our findings demonstrate that DPP6, in addition to its role as a Kv4 partner regulating dendritic excitability in hippocampal CA1 pyramidal neurons, has an important developmental role by promoting dendritic filopodia formation and stability, subsequently affecting synapse development and function. DPP6 is important for filopodia formation and stability We found that labelled DPP6 localizes to dendritic filopodia and spines ( Supplementary Fig. S1 ), suggesting a potential role in synaptic development. To investigate this possibility, we first measured dendritic filopodia formation in the hippocampal neurons cultured from P0 wild type (WT) and DPP6-KO mice. The density of immature dendritic filopodia at DIV3 in cultured hippocampal neurons obtained from DPP6-KO mice was significantly decreased, to about 45% of that found for WT ( Fig. 1a,b ; P <0.05, unpaired Student’s t -test). In a second experiment, we expressed either green fluorescent protein (GFP) or GFP-tagged DPP6 (DPP6-GFP) in P0 DPP6-KO mouse hippocampal neurons and counted the number of immature dendritic filopodia at DIV3. DPP6-GFP-expressing neurons showed a significantly increased density of immature dendritic filopodia compared with the GFP control demonstrating a specific role for DPP6 in regulating filopodia number ( Fig. 1c,d ; P <0.05, unpaired Student’s t -test). We also measured the density of filopodia in identified axons (Tau-1 positive) in cultured neurons at DIV3. Unlike our results for immature dendritic filopodia, we found no significant difference in the number of axonal filopodia between DPP6-KO and WT neurons (WT=1.81±0.16 filopodia per 20 μm axon length, n= 64; DPP6-KO=1.40±0.13 filopodia per 20 μm axon length, n= 85, P >0.05, unpaired Student’s t -test). Although the density of filopodia in the identified dendrites of DPP6-KO-cultured neurons is significantly decreased compared with WT, we did not find a significant difference between the density of dendritic branches of DIV3 WT and DPP6-KO-cultured neurons (WT=0.08±0.02 branches per 20 μm, n= 44; DPP6-KO=0.07±0.01 branches per 20 μm, n= 77, P >0.05, unpaired Student’s t -test). 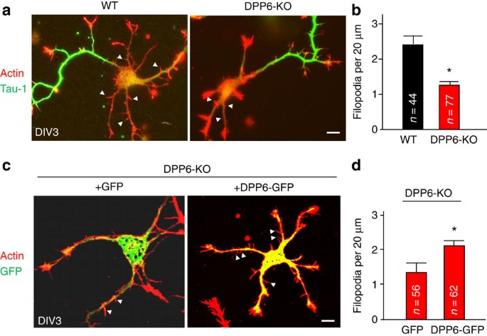Figure 1: Dendritic filopodia formation is reduced in DPP6-KO hippocampal neurons and rescued by DPP6 expression. (a,b) DIV3 WT or DPP6-KO hippocampal neurons visualized for actin filaments with TRITC-phalloidin (1:1000, Sigma) and for axons with marker Tau-1 (1:1000, Millipore). The density of immature dendritic filopodia (arrowheads) is decreased in the DPP6-KO neurons (n=77) compared with the WT (n=44). (c,d) DIV3 DPP6-KO hippocampal neurons expressing either GFP control or DPP6-GFP cultured for 3 days, and visualized for actin filaments with TRITC-phalloidin. The density of filopodia is increased in the DPP6-KO neurons that expressed DPP6-GFP (n=62) compared with the GFP controls (n=56). Scale bars, 10 μm. Error bars represent the mean±s.e.m. *P<0.05, unpaired Student’st-test. Figure 1: Dendritic filopodia formation is reduced in DPP6-KO hippocampal neurons and rescued by DPP6 expression. ( a , b ) DIV3 WT or DPP6-KO hippocampal neurons visualized for actin filaments with TRITC-phalloidin (1:1000, Sigma) and for axons with marker Tau-1 (1:1000, Millipore). The density of immature dendritic filopodia (arrowheads) is decreased in the DPP6-KO neurons ( n= 77) compared with the WT ( n= 44). ( c , d ) DIV3 DPP6-KO hippocampal neurons expressing either GFP control or DPP6-GFP cultured for 3 days, and visualized for actin filaments with TRITC-phalloidin. The density of filopodia is increased in the DPP6-KO neurons that expressed DPP6-GFP ( n= 62) compared with the GFP controls ( n= 56). Scale bars, 10 μm. Error bars represent the mean±s.e.m. * P <0.05, unpaired Student’s t -test. Full size image These results, showing a role for DPP6 in regulating filopodia number, could indicate either an effect on filopodia formation, the stability of filopodia once formed, or both. To determine this, we performed live imaging experiments to monitor filopodia in DIV3 hippocampal neurons from WT and DPP6-KO mice ( Fig. 2 ). First we measured the mean lifetime of existing filopodia over 1 h at 30-s intervals. Fig. 2a,b shows that filopodia in WT neurons are very stable, with~75% of 78 total filopodia lasting the full 60 min of time-lapse recording. In DPP6-KO neurons, however, only ~57% of 80 total filopodia lasted the full hour. Next, we measured the effect of transfecting either GFP or DPP6-GFP into DPP6-KO P0 hippocampal neurons. Results showed that filopodia in DPP6-GFP-expressing neurons were more stable (~70% survival for 1 h) compared with the GFP control (~59% survival, Fig. 2c,d ). This rescue of filopodia stability in DPP6-KO neurons to WT levels by DPP6-GFP expression suggests a fundamental role for the DPP6 protein in maintaining filopodia in developing hippocampal neurons. 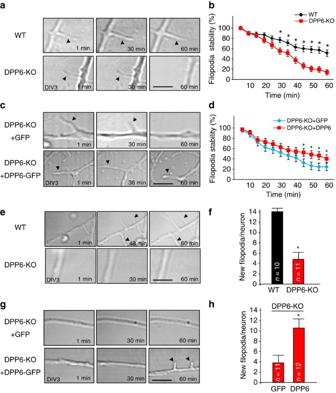Figure 2: Dendritic filopodia are less stable and fewer new filopodia are initiated in DPP6-KO neurons than in WT hippocampal neurons. The lifetimes of individual filopodia were assayed for 1 hr in phase-contrast, time-lapse sequences of transfected neurons (n=10 neurons for each condition). (a,b) Images of WT and DPP6-KO neurons showing filopodia (arrowheads). The graph shows the percentage of stable (lifetime of at least 60 min) filopodia for WT and DPP6-KO neurons. (c,d) Images of DIV3 DPP6-KO neurons expressing either GFP or DPP6-GFP. Arrowheads point out filopodia. The graph shows the percentage of stable (lifetime of at least 60 min) filopodia for each condition. (e,f) DPP6-KO mice showed less initiation of new filopodia (arrow) over the course of 1-hr recordings compared with WT. (g,h) Expression of DPP6 in DPP6-KO mice increased the number of filopodia initiated. Scale bars, 10 μm. Error bars represent the mean±s.e.m. *P<0.05, unpaired Student’st-test. Figure 2: Dendritic filopodia are less stable and fewer new filopodia are initiated in DPP6-KO neurons than in WT hippocampal neurons. The lifetimes of individual filopodia were assayed for 1 hr in phase-contrast, time-lapse sequences of transfected neurons ( n= 10 neurons for each condition). ( a , b ) Images of WT and DPP6-KO neurons showing filopodia (arrowheads). The graph shows the percentage of stable (lifetime of at least 60 min) filopodia for WT and DPP6-KO neurons. ( c , d ) Images of DIV3 DPP6-KO neurons expressing either GFP or DPP6-GFP. Arrowheads point out filopodia. The graph shows the percentage of stable (lifetime of at least 60 min) filopodia for each condition. ( e , f ) DPP6-KO mice showed less initiation of new filopodia (arrow) over the course of 1-hr recordings compared with WT. ( g , h ) Expression of DPP6 in DPP6-KO mice increased the number of filopodia initiated. Scale bars, 10 μm. Error bars represent the mean±s.e.m. * P <0.05, unpaired Student’s t -test. Full size image In these live imaging studies, we also counted the number of new filopodia initiated during the 1 h recording ( Fig. 2e,f ). We found DPP6-KO neurons to produce about 60% fewer filopodia than WT ( P <0.05, unpaired Student’s t -test). In DPP6-GFP-expressing DPP6-KO hippocampal neurons, we found that DPP6-GFP increased the initiation of filopodia about threefold compared with the GFP control, nearly restoring the rate of filopodia formation to WT levels ( Fig. 2g,h ; P <0.05, unpaired Student’s t -test). Taken together, the live imaging measurements suggest that the decreased density of filopodia in DPP6-KO hippocampal neurons is due to a combination of both decreased stability and initiation of filopodia by DPP6. Spine density is reduced in developing DPP6-KO neurons As filopodia can transform into spines [22] , we looked for a corresponding effect on spine number at a later developmental stage. To detect and count spines in dendrites, cultures were immunostained for mitogen-activated protein 2 to highlight the dendritic arbor, and PSD-95 to visualize spines at postsynaptic sites (see Methods). 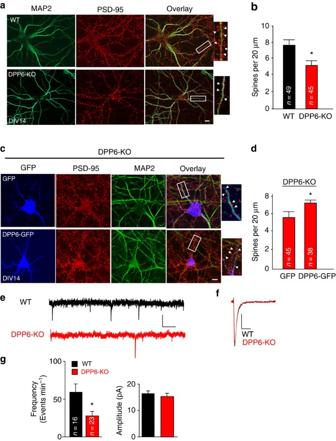Figure 3: Dendritic spine formation is reduced in DPP6-KO hippocampal neurons. (a,b) P0 WT or DPP6-KO neurons were cultured until DIV14, then immunostained with MAP2 (green, 1:1000, Chemicon) to highlight the dendritic arbor, and PSD-95 (red, 1:200, NeuroMab) as a spine marker. Inset in the right-hand panel is an enlargement of the boxed area. Arrowheads indicate examples of spines. Graph showing that the density of spines in DPP6-KO mice hippocampal neurons (n=45) is decreased compared with WT (n=49). Scale bar, 10 μm. (c,d) DIV14 DPP6-KO hippocampal neurons expressing either GFP or DPP6-GFP. Inset in the right-hand panel is an enlargement of the boxed area. Arrowheads indicate examples of spines. Graph shows that DPP6-GFP (n=38) increased spine density compared with GFP controls (n=45). Scale bar, 10 μm. mEPSC frequency, but not amplitude, is decreased in DPP6-KO hippocampal neurons. (e,f) Sample mEPSC traces from WT and DPP6-KO cultured hippocampal neurons recorded at DIV14 and 15. Scale bars: 10 pA, 250 ms (e) and 4 pA, 20 ms (f). (g) Average mini frequency is decreased in DPP6-KO (n=23) versus WT (n=16) cultured hippocampal neurons, whereas amplitude is not affected. Error bars represent the mean±s.e.m. *P<0.05, unpaired Student’st-test. Figure 3a shows images of cultured WT and DPP6-KO hippocampal neurons at DIV14. The density of the spines (number per 20 μm length) was reduced in DPP6-KO neurons ~30% compared with those from WT mice ( Fig. 3b ; P <0.05, unpaired Student’s t -test). As found for dendritic filopodia ( Figs 1 and 2 ), expression of DPP6-GFP in DPP6-KO mouse P0 hippocampal neurons enhanced spine density compared with GFP controls when measured at DIV 14 ( Fig. 3c,d ; P <0.05, unpaired Student’s t -test). To determine the functional impact of spine density decrease in DPP6-KO neurons, we measured miniature excitatory synaptic currents in DIV14-cultured WT and DPP6-KO neurons. While no differences between the two groups were found for mEPSC amplitude, mEPSC frequency was significantly decreased in DPP6-KO neurons ( Fig. 3e,g , P <0.05, unpaired Student’s t -test). Therefore, in addition to regulating filopodia number early in development, DPP6 subsequently impacts spine formation and synapse number in the hippocampal neurons. Figure 3: Dendritic spine formation is reduced in DPP6-KO hippocampal neurons. ( a , b ) P0 WT or DPP6-KO neurons were cultured until DIV14, then immunostained with MAP2 (green, 1:1000, Chemicon) to highlight the dendritic arbor, and PSD-95 (red, 1:200, NeuroMab) as a spine marker. Inset in the right-hand panel is an enlargement of the boxed area. Arrowheads indicate examples of spines. Graph showing that the density of spines in DPP6-KO mice hippocampal neurons ( n= 45) is decreased compared with WT ( n= 49). Scale bar, 10 μm. ( c , d ) DIV14 DPP6-KO hippocampal neurons expressing either GFP or DPP6-GFP. Inset in the right-hand panel is an enlargement of the boxed area. Arrowheads indicate examples of spines. Graph shows that DPP6-GFP ( n= 38) increased spine density compared with GFP controls ( n= 45). Scale bar, 10 μm. mEPSC frequency, but not amplitude, is decreased in DPP6-KO hippocampal neurons. ( e , f ) Sample mEPSC traces from WT and DPP6-KO cultured hippocampal neurons recorded at DIV14 and 15. Scale bars: 10 pA, 250 ms ( e ) and 4 pA, 20 ms ( f ). ( g ) Average mini frequency is decreased in DPP6-KO ( n= 23) versus WT ( n= 16) cultured hippocampal neurons, whereas amplitude is not affected. Error bars represent the mean±s.e.m. * P <0.05, unpaired Student’s t -test. Full size image Developmental effects of DPP6 knockdown To see if DPP6’s role in regulating dendritic spine formation impacted synaptogenesis, we used RNA interference against DPP6 in the hippocampal neuron cultures over a period of rapid synapse formation and a decrease in dendritic filopodia density. E18 rat hippocampal neurons were transfected with either RNA interference targeting DPP6 (‘siDPP6’) [23] or control RNA interference (siCtrl) at plating. As a control, we measured the effect of siDPP6 expression on filopodia number in neurons cultured from DPP6-KO mice. Neither siDPP6 nor siCtrl affected the number of filopodia in DPP6-KO neurons (DPP6-KO+siCtrl=1.49±0.24 filopodia per 20 μm, n= 12; DPP6-KO+siDPP6=1.35±0.26 filopodia per 20 μm, n= 14, P >0.05, unpaired Student’s t -test). At DIV7, 14 and 21 cultured neurons were fixed and immunostained with mitogen-activated protein 2 to highlight the dendritic arbor, and with phalloidin to highlight actin-based protrusions. To measure the density of synapses, we co-labelled neurons with the presynaptic marker synaptophysin and the post-synapse marker PSD-95. Puncta where synaptophysin and PSD-95 labelling overlapped were counted as synapses. To determine the effect of DPP6 knockdown on the formation of filopodia, spines and synaptogenesis, we detected and counted the density of filopodia, spines and synapses in maturing WT hippocampal neurons and transfected neurons either with siCtrl-GFP or siDPP6-GFP. WT hippocampal neuronal cultures displayed a progressive decrease in the density of filopodia between DIV7 and DIV21, and a corresponding increase in the density of spines and synapses during maturation ( Supplementary Fig. S2 ). In siDPP6-expressing neurons, we found the density of filopodia was significantly reduced by ~42% at DIV7 and ~30% at DIV14 compared with siCtrl ( Fig. 4a,b,e ; P <0.05, unpaired Student’s t -test). The number of filopodia was negligible in both groups by DIV21 ( Fig. 4c,e ). We also found siDPP6 to cause a corresponding decrease in the spine density by ~40% at DIV14, and ~50% at DIV21 compared with siCtrl ( Fig. 4b,c,f ; P <0.05, unpaired Student’s t -test) while the density of synapses was reduced by ~20% at DIV14 and 40% in DIV21 neurons expressing siDPP6 compared with siCtrl ( Fig. 4c,g ; P <0.05, unpaired Student’s t -test). Accordingly, mEPSC frequency was reduced in siDPP6-expressing neurons compared with control (siCtrl=105.7±28.1 events min −1 , n= 20; siDPP6=43.3±9.0 events min −1 , n= 17, P <0.05, unpaired Student’s t -test). No difference in mEPSC amplitude was found, however (siCtrl=15.4±1.3 pA, n= 20; siDPP6=13.8±1.5 pA, n= 17, P >0.05, unpaired Student’s t -test). Moreover, expression of DPP6-GFP in mature DPP6-KO neurons increased the number of spines compared with control DPP6-KO neurons expressing only GFP controls (DPP6-KO+GFP=5.26±0.23 spines per 20 μm, n= 45; DPP6-KO+DPP6-GFP=7.11±0.31 spines per 20 μm, n= 38, P >0.05, unpaired Student’s t -test). These results show that DPP6 is important in regulating the development of synapses in hippocampal neurons. 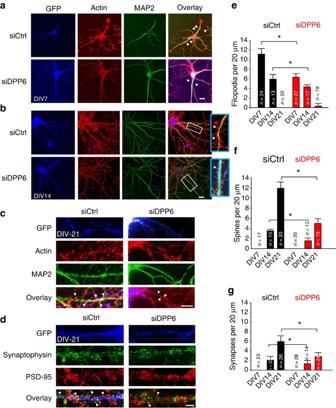Figure 4: DPP6 knockdown causes a reduction in filopodia and synapses during development in the hippocampal cultured neurons. (a–c) Fixed hippocampal neurons were immunostained for F-actin (red), to visualize filopodia and spines and MAP2 (green) to highlight the dendritic arbor and GFP (blue). (a) Arrowheads indicate examples of filopodia; (b,c) arrowheads indicate examples of spines. (d) Fixed hippocampal neurons were immunostained for PSD-95 (red), to visualize postsynaptic sites and synaptophysin (green) to highlight the presynaptic boutons and GFP (blue). Overlapping puncta of PSD-95 and synaptophysin were considered to be synapses. Examples shown here are DIV21. Arrowheads indicate examples of synapses. Scale bars, 10 μm. (e) Graph comparing the number of filopodia per 100 μm dendrite length for siCtrl (n=24, 13, 20) and siDPP6 (n=27, 17, 19) expressing hippocampal neurons at DIV7, 14 and 21, respectively. (f) Graph comparing the number of spines per 20 μm dendrite length for siCtrl (n=17, 13, 20) and siDPP6 (n=20, 17, 19) expressing hippocampal neurons at DIV7, 14 and 21, respectively. (g) Graph comparing the number of synapses per 20 μm dendrite length for siCtrl (n=23, 23, 26) and siDPP6 (n=28, 14, 24) expressing hippocampal neurons at DIV7, 14 and 21, respectively. Error bars represent the mean±s.e.m. *P<0.05, unpaired Student’st-test. Figure 4: DPP6 knockdown causes a reduction in filopodia and synapses during development in the hippocampal cultured neurons. ( a – c ) Fixed hippocampal neurons were immunostained for F-actin (red), to visualize filopodia and spines and MAP2 (green) to highlight the dendritic arbor and GFP (blue). ( a ) Arrowheads indicate examples of filopodia; ( b , c ) arrowheads indicate examples of spines. ( d ) Fixed hippocampal neurons were immunostained for PSD-95 (red), to visualize postsynaptic sites and synaptophysin (green) to highlight the presynaptic boutons and GFP (blue). Overlapping puncta of PSD-95 and synaptophysin were considered to be synapses. Examples shown here are DIV21. Arrowheads indicate examples of synapses. Scale bars, 10 μm. ( e ) Graph comparing the number of filopodia per 100 μm dendrite length for siCtrl ( n= 24, 13, 20) and siDPP6 ( n= 27, 17, 19) expressing hippocampal neurons at DIV7, 14 and 21, respectively. ( f ) Graph comparing the number of spines per 20 μm dendrite length for siCtrl ( n= 17, 13, 20) and siDPP6 ( n= 20, 17, 19) expressing hippocampal neurons at DIV7, 14 and 21, respectively. ( g ) Graph comparing the number of synapses per 20 μm dendrite length for siCtrl ( n= 23, 23, 26) and siDPP6 ( n= 28, 14, 24) expressing hippocampal neurons at DIV7, 14 and 21, respectively. Error bars represent the mean±s.e.m. * P <0.05, unpaired Student’s t -test. Full size image DPP6 effects are independent of Kv4.2 DPP6 is important in regulating Kv4.2 dendritic expression and function [13] . To see if the effects of DPP6 loss on synaptic development involved its role as a Kv4.2 auxiliary subunit, we repeated the above experiments using DIV3 Kv4.2-KO cultured neurons. However, unlike for DPP6-KO neurons, results showed that the density of filopodia in the axon and immature dendrites are not significantly different between Kv4.2-KO and WT neurons ( Fig. 5 ; for dendritic filopodia, WT=2.33±0.24 filopodia per 20 μm, n= 44; Kv4.2-KO=2.11±0.19 filopodia per 20 μm, n= 45, P >0.05; for filopodia in the axon, WT=1.81±0.16 filopodia per 20 μm, n= 64; Kv4.2-KO=1.87±0.32 filopodia per 20 μm, n= 58, P >0.05, unpaired Student’s t -tests). We also observed no differences in the number of immature dendritic branches (WT=0.08±0.02 branches per 20 μm, n= 44; Kv4.2-KO=0.09±0.01 branches per 20 μm, n= 45, P >0.05, unpaired Student’s t -test). At DIV14, we found that the number of spines are unchanged in Kv4.2-KO neurons compared with WT (WT=7.66±0.29 spines per 20 μm, n= 49; Kv4.2-KO=6.88±0.27 spines per 20 μm, n= 47, P >0.05, unpaired Student’s t -test) and neither mEPSC frequency (WT=58.2±11.8 events min −1 , n= 25; Kv4.2-KO=43.3±8.9 events min −1 , n= 25, P >0.05, unpaired Student’s t -test) nor amplitude (WT=16.4±0.9 pA, n= 25; Kv4.2-KO=15.7±1.2 pA, n= 25, P >0.05, unpaired Student’s t -test) differed. Therefore, we conclude that the effect of DPP6 on filopodia formation and stability occurs independent of its role as a Kv4.2 auxiliary subunit. 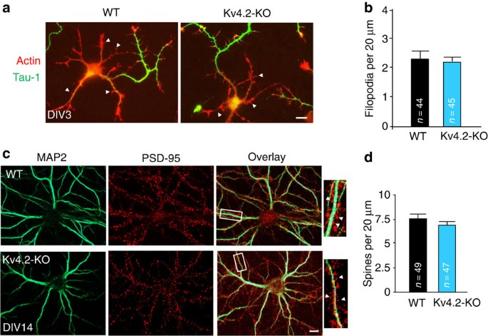Figure 5: Dendritic filopodia and spine density unaltered in Kv4.2-KO hippocampal neurons. (a,b) DIV3 WT or Kv4.2-KO hippocampal neurons visualized for actin filaments with TRITC-phalloidin (1:1000, Sigma) and for axons with marker Tau-1 (1:1000, Millipore). The density of filopodia (arrowheads) is not significantly different in Kv4.2-KO neurons compared with WT (P>0.05). (c,d) DIV14 WT or Kv4.2-KO neurons were cultured and immunostained with MAP2 (green, 1:1000, Chemicon) to highlight the dendritic arbor, and PSD-95 (red, 1:200, NeuroMab) as a spine marker. Inset in the right-hand panel is an enlargement of the boxed area. Arrowheads indicate examples of spines. Graph showing that the density of spines in Kv4.2-KO mouse hippocampal neurons is not changed compared with WT. Scale bars, 10 μm. Error bars represent the mean±s.e.m. Figure 5: Dendritic filopodia and spine density unaltered in Kv4.2-KO hippocampal neurons. ( a , b ) DIV3 WT or Kv4.2-KO hippocampal neurons visualized for actin filaments with TRITC-phalloidin (1:1000, Sigma) and for axons with marker Tau-1 (1:1000, Millipore). The density of filopodia (arrowheads) is not significantly different in Kv4.2-KO neurons compared with WT ( P >0.05). ( c , d ) DIV14 WT or Kv4.2-KO neurons were cultured and immunostained with MAP2 (green, 1:1000, Chemicon) to highlight the dendritic arbor, and PSD-95 (red, 1:200, NeuroMab) as a spine marker. Inset in the right-hand panel is an enlargement of the boxed area. Arrowheads indicate examples of spines. Graph showing that the density of spines in Kv4.2-KO mouse hippocampal neurons is not changed compared with WT. Scale bars, 10 μm. Error bars represent the mean±s.e.m. Full size image Consequences of DPP6-deficiency in adult neurons To determine if the developmental effects described above are functionally relevant into adulthood, we used biocytin staining to isolate single CA1 pyramidal neurons from both 6–8-week-old WT and DPP6-KO mice. Compared with WT controls, pyramidal cells from adult DPP6-KO mice exhibited a significant reduction in spine density in both apical and basal dendritic locations ( Fig. 6a,b ). When the data were subdivided into distinct parts of the apical dendrite, it was apparent that DPP6-KO mouse spine density decreased dramatically (~52%) in distal dendrites (~240 μm) compared with WT ( n= 10 for DPP6-KO, n= 10 for WT, P <0.05, unpaired Student’s t -test), whereas only a small reduction (~15%) in spine number was observed in proximal dendrites (~40 μm, n= 10 for DPP6-KO, n= 10 for WT). 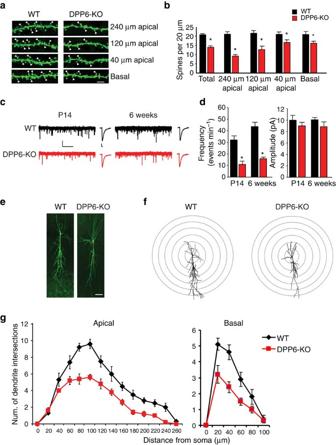Figure 6: DPP6 loss affects the excitatory synaptic function and dendritic branch complexity in adult hippocampal CA1 pyramidal neurons. (a) Representative dendritic spine (arrowheads) images of CA1 neurons from WT and DPP6-KO mice at specific distances. Scale bar, 5 μm. (b) Quantification of spine number (n=10 for DPP6-KO,n=10 for WT). (c) Representative mEPSC recordings from WT and DPP6-KO CA1 hippocampal pyramidal neurons from P14 (left traces) and 6–8-week-old mice (right traces). Sweep scale bar, 10 pA, 20 ms. Average mEPSC scale bar, 1 pA, 10 ms. (d) mEPSC frequency (P14 mice WTn=8, DPP6-KOn=7; adult micen=10 each WT and DPP6-KO), but not peak amplitude in P14 and adult mice (P>0.1) is altered in DPP6-KO neurons. Error bars represent the mean±s.e.m. (e) A simpler dendritic branching pattern is observed in neurons from DPP6-KO mice. Images showing biocytin-filled neurons labelled with Alexa-488 conjugated streptavidin in 6–8-week-old WT and DPP6-KO mice. Scale bar, 50 μm. (f) Traced confocal stack images from WT and DPP6-KO mice CA1 hippocampal neurons. (g) Number of dendritic intersections of WT and DPP6-KO neurons plotted versus distance for apical and basal dendrites (n=10 for WT,n=10 for DPP6-KO,P<0.05, unpaired Student’st-test). Error bars represent the mean±s.e.m. *P<0.05, unpaired Student’st-test. Figure 6: DPP6 loss affects the excitatory synaptic function and dendritic branch complexity in adult hippocampal CA1 pyramidal neurons. ( a ) Representative dendritic spine (arrowheads) images of CA1 neurons from WT and DPP6-KO mice at specific distances. Scale bar, 5 μm. ( b ) Quantification of spine number ( n= 10 for DPP6-KO, n= 10 for WT). ( c ) Representative mEPSC recordings from WT and DPP6-KO CA1 hippocampal pyramidal neurons from P14 (left traces) and 6–8-week-old mice (right traces). Sweep scale bar, 10 pA, 20 ms. Average mEPSC scale bar, 1 pA, 10 ms. ( d ) mEPSC frequency (P14 mice WT n= 8, DPP6-KO n= 7; adult mice n= 10 each WT and DPP6-KO), but not peak amplitude in P14 and adult mice ( P >0.1) is altered in DPP6-KO neurons. Error bars represent the mean±s.e.m. ( e ) A simpler dendritic branching pattern is observed in neurons from DPP6-KO mice. Images showing biocytin-filled neurons labelled with Alexa-488 conjugated streptavidin in 6–8-week-old WT and DPP6-KO mice. Scale bar, 50 μm. ( f ) Traced confocal stack images from WT and DPP6-KO mice CA1 hippocampal neurons. ( g ) Number of dendritic intersections of WT and DPP6-KO neurons plotted versus distance for apical and basal dendrites ( n= 10 for WT, n= 10 for DPP6-KO, P <0.05, unpaired Student’s t -test). Error bars represent the mean±s.e.m. * P <0.05, unpaired Student’s t -test. Full size image To determine if this loss of spines leads to functional impairments, we performed electrophysiological recordings from WT and DPP6-KO adult acute hippocampal slices. Genetic loss of DPP6 resulted in a significant decrease of mEPSC frequency in both P14 young mice ( Fig. 6c,d ; WT n= 8; DPP6-KO n= 7; P <0.05, unpaired Student’s t -test) and adult mice compared with WT ( Fig. 6c,d ; WT n= 6; DPP6-KO n= 7; P <0.05, unpaired Student’s t -test). mEPSC amplitude was not significantly affected by DPP6 loss at either developmental stage ( Fig. 6c,d ; P14 amplitude for WT n= 8, DPP6-KO n= 7; adult amplitude for WT n= 6, DPP6-KO n= 7; P >0.1). No differences were found between genotypes in paired-pulse facilitation experiments ( Supplementary Fig. S3 ) indicating a postsynaptic effect of DPP6 loss. Taken together, the reduction of mEPSC frequency but not amplitude, along with the lack of paired pulse facilitation change suggests that DPP6-KO mice have fewer functional excitatory synapses in CA1 neuron dendrites. We therefore investigated dendritic morphology in the biocytin-stained hippocampal CA1 pyramidal neurons in both WT and DPP6-KO mice ( Fig. 6e,g ). Sholl analysis revealed a simpler dendritic branching pattern in neurons from DPP6-KO mice compared with WT controls ( Fig. 6f,g ). We found in DPP6-KO mice, less dendritic intersections at locations greater than 40 μm from the soma throughout the dendritic tree compared with WT ( Fig. 6g ; n= 10 for DPP6, n= 10 for WT, P <0.05, unpaired Student’s t -test). In DPP6-KO neurons, apical dendrite trunk length was not different from WT (WT=232.1±17.0 μm, DPP6-KO=225.1±19.3 μm, n= 10, P >0.05), but the total apical dendritic length of DPP6-KO is significantly decreased (WT=781.6±46.4 μm, DPP6=488.6±51.0 μm, n= 10, P <0.05, unpaired Student’s t -test). The decrease in functional excitatory synapses in DPP6-KO CA1 neurons compared with WT may then be accounted by their sparse dendritic arbor as well as their reduced spine density per unit length of remaining apical dendrites. This finding differs from that reported above for DIV3 DPP6-KO neurons where we did not find a difference from WT in the number of dendritic branches at this young stage, indicating a developmental impact of DPP6 on branch complexity. As described above ( Fig. 5 ), we determined that DPP6 acts independent of its role as a Kv4.2 auxiliary subunit in developing neurons, as filopodia formation and stability were not affected in Kv4.2-KO neurons. Consequently, in adult mice, we also found no effect of Kv4.2-KO on dendritic branching compared with WT ( Supplementary Fig. S4 ). Mechanism of DPP6 effects on filopodia Our results indicate that DPP6 has a role in regulation of synaptic development and function including filopodia formation and stability. Protrusion of filopodia involves the reorganization of the actin cytoskeleton. To understand the molecular mechanisms underlying DPP6’s effects on synaptic development, we immunoprecipitated DPP6 from lysates of the hippocampal neurons to identify DPP6 interacting proteins ( Fig. 7a ). Mass spectrometry of bands that were immunoprecipitated from WT but not DPP6-KO neurons led to the identification of Myosin-X as a DPP6 interacting protein. Myosin-X is an unconventional myosin known to be important in the formation and elongation of filopodia [24] . Myosin-X is also thought to transport cargo molecules within filopodia and provides a motor-base link between integrins and the cytoskeleton [25] . 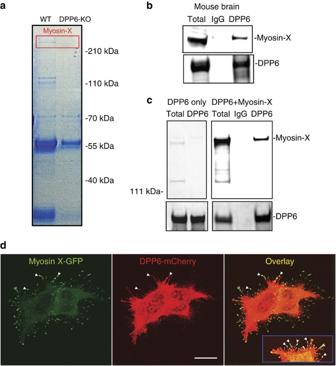Figure 7: DPP6 co-immunoprecipitates with Myosin-X. (a) WT and DPP6-KO DIV14 neuron lysates were pulled down with a DPP6 antibody, and separated by 4–12% SDS–PAGE. The gel is stained with Coomassie blue. Red box shows loss of Myosin-X pulldown in DPP6-KO mice. Scale bar, 50 μm. (b) Native co-IP from mouse brain shows that endogenous DPP6 interacts with Myosin-X. IgG as nonspecific control. (c) DPP6 binds with Myosin-X in COS7 cells co-transfected with DPP6 and Myosin-X in a co-IP assay. A DPP6 antibody was used for pull-down and lysates are probed with an anti-Myosin-X antibody (1:4000, Sigma) or anti-DPP6 antibody (1:2000, Abcam), then visualized by anti-rabbit Alexa Fluor 680 and anti-rabbit Alexa Fluor 800 secondary antibody, respectively. Scale bar, 50 μm. (d) Images of Myosin-X-GFP (green) and DPP6-Cherry (red) expressed in COS7 cells, showing their localization at the tip of filopodia (yellow, arrowheads, overlapping signals). Scale bar, 10 μm. Figure 7: DPP6 co-immunoprecipitates with Myosin-X. ( a ) WT and DPP6-KO DIV14 neuron lysates were pulled down with a DPP6 antibody, and separated by 4–12% SDS–PAGE. The gel is stained with Coomassie blue. Red box shows loss of Myosin-X pulldown in DPP6-KO mice. Scale bar, 50 μm. ( b ) Native co-IP from mouse brain shows that endogenous DPP6 interacts with Myosin-X. IgG as nonspecific control. ( c ) DPP6 binds with Myosin-X in COS7 cells co-transfected with DPP6 and Myosin-X in a co-IP assay. A DPP6 antibody was used for pull-down and lysates are probed with an anti-Myosin-X antibody (1:4000, Sigma) or anti-DPP6 antibody (1:2000, Abcam), then visualized by anti-rabbit Alexa Fluor 680 and anti-rabbit Alexa Fluor 800 secondary antibody, respectively. Scale bar, 50 μm. ( d ) Images of Myosin-X-GFP (green) and DPP6-Cherry (red) expressed in COS7 cells, showing their localization at the tip of filopodia (yellow, arrowheads, overlapping signals). Scale bar, 10 μm. Full size image For further confirmation, on DPP6–Myosin-X interaction, we found that endogenous DPP6 and Myosin-X co-immunoprecipitate in lysates from mouse brain ( Fig. 7b ). DPP6 and Myosin-X also co-immunoprecipitated when transfected into COS7 cells ( Fig. 7c ). As one of the most intriguing features of Myosin-X is its localization at the tips of filopodia [26] , [27] , we also tested if DPP6 is present in this location. As shown in Fig. 8d , DPP6 and Myosin-X are both present at the tips of filopodia ( Fig. 7d ). HEK cells, co-expressing the membrane protein marker, membrane-mCherry, along with DPP6-GFP showed clear colocalization suggesting membrane expression of DPP6-GFP ( Supplementary Fig. S5 ). 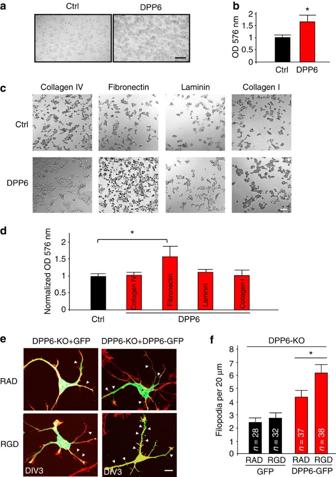Figure 8: DPP6 promotes cell adhesion and binds with ECM fibronectin. Transfected COS7 cells were plated on 96-well dishes coated with poly-L-lysine (a,b) or coated with ECM proteins (collagen IV, fibronectin, laminin or collagen I, respectively) (c,d) for 1 h. Non-adherent cells were washed off and adherent cells were assayed by crystal violet staining. Expression of DPP6 significantly increased COS7 cell adhesion to the substratum poly-L-lysine compared with the control cells (P<0.001, unpaired Student’st-test) (a,b). Graphs shows mean OD and standard error (n=4 experiments). COS7 cells expressing DPP6 showed significantly improved cell attachment to Fibronectin, but not to Collagen IV, Laminin or Collagen I, compared with the control cells (P<0.001, unpaired Student’st-test) (c,d). Graphs show mean OD and standard error (n=3 experiments). (e,f) Dendritic filopodia are enhanced by RGD peptides in DIV3 DPP6-GFP-expressing hippocampal neurons. (e) DPP6-KO hippocampal neurons either expressed GFP (left) or DPP6-GFP (right). DIV3 neurons were treated with control RAD or RGD peptides (250 μM, 60 min), fixed and visualized for actin filaments with TRITC-phalloidin (1:1000, Sigma). Arrowheads point out filopodia. (f) The density of filopodia in GFP-expressing neurons with RDG treatment in DPP6-KO mice was slightly increased compared with control RAD treatment (n=28 for RAD,n=32 for RGD treatment,P>0.05, unpaired Student’st-test), but in DPP6-KO neurons expressing DPP6-GFP, the density of filopodia is significantly increased with RGD treatment compared with the control (n=37 for RAD,n=38 for RGD treatment,P<0.05, unpaired Student’st-test). Scale bar, 10 μm. Error bars represent the mean±s.e.m. Figure 8: DPP6 promotes cell adhesion and binds with ECM fibronectin. Transfected COS7 cells were plated on 96-well dishes coated with poly-L-lysine ( a , b ) or coated with ECM proteins (collagen IV, fibronectin, laminin or collagen I, respectively) ( c , d ) for 1 h. Non-adherent cells were washed off and adherent cells were assayed by crystal violet staining. Expression of DPP6 significantly increased COS7 cell adhesion to the substratum poly-L-lysine compared with the control cells ( P <0.001, unpaired Student’s t -test) ( a , b ). Graphs shows mean OD and standard error ( n= 4 experiments). COS7 cells expressing DPP6 showed significantly improved cell attachment to Fibronectin, but not to Collagen IV, Laminin or Collagen I, compared with the control cells ( P <0.001, unpaired Student’s t -test) ( c , d ). Graphs show mean OD and standard error ( n= 3 experiments). ( e , f ) Dendritic filopodia are enhanced by RGD peptides in DIV3 DPP6-GFP-expressing hippocampal neurons. ( e ) DPP6-KO hippocampal neurons either expressed GFP (left) or DPP6-GFP (right). DIV3 neurons were treated with control RAD or RGD peptides (250 μM, 60 min), fixed and visualized for actin filaments with TRITC-phalloidin (1:1000, Sigma). Arrowheads point out filopodia. ( f ) The density of filopodia in GFP-expressing neurons with RDG treatment in DPP6-KO mice was slightly increased compared with control RAD treatment ( n= 28 for RAD, n= 32 for RGD treatment, P >0.05, unpaired Student’s t -test), but in DPP6-KO neurons expressing DPP6-GFP, the density of filopodia is significantly increased with RGD treatment compared with the control ( n= 37 for RAD, n= 38 for RGD treatment, P <0.05, unpaired Student’s t -test). Scale bar, 10 μm. Error bars represent the mean±s.e.m. Full size image DPP6 induces filopodia formation through cell adhesion As with other DPPs, the extracellular domain of DPP6 consists of a β-propeller and an α/β-hydrolase domain [15] . β-propellers provide excellent platforms for protein–protein interactions, and in DPPIV (also termed CD26) the extracellular domain binds to components of the ECM like collagen, fibronectin and integrin β1 [16] , [17] , [28] . DPP6 has approximately 50% similarity to CD26 [21] and also has a cysteine-rich domain that may bind to components of the ECM function in cell adhesion. We investigated the effects of DPP6 transfection on adhesion of COS7 cells to the culture substratum poly-L-lysine. We found that COS7 co-expressed with DPP6-enhanced cell adhesion about twofold compared with the control cells transfected with vector only ( Fig. 8a,b ; P <0.05, unpaired Student’s t -test), indicating that DPP6 promotes cell adhesion to the substratum. Integrins form a large family of heterodimeric (α/β-subunits) membrane-spanning ECM receptors [29] , [30] , which bind to an arginine-glycine-aspartate (RGD) motif found in many ECM proteins. As this short peptide sequence is able to interact with integrin receptors on the cell surface by itself, the RGD motif has frequently been introduced into various polymeric materials to enhance their cell adhesive abilities for use in tissue engineering. To determine whether DPP6 has a role in cell adhesion by binding to RGD motifs in ECM proteins, we mimicked the effects of ECM on integrin signalling in the cultured hippocampal neurons by applying an RGD-containing peptide and then examined its effects on filopodia formation. The cultured P0 DPP6-KO hippocampal neurons expressing either GFP or DPP6-GFP were treated at DIV3 with either control RAD or RGD-containing peptides (250 μM, 60 min). The neurons were then fixed and their actin filaments visualized with TRITC-phalloidin. We counted the number of filopodia per dendrite length and found that, upon RGD treatment, the density of filopodia is slightly but not significantly increased in DPP6-KO neurons compared with the control RAD peptides treatment ( Fig. 8e,f P >0.1). However, with the same RGD treatment in DPP6-GFP-expressing DPP6-KO neurons, filopodia were significantly increased by ~40% compared with the control RAD ( P <0.05, unpaired Student’s t -test). These results are compatible with that of Shi and Ethell [31] who showed that RGD treatment induced elongation of existing dendritic spines and promoted formation of new filopodia, suggesting that the RGD peptide acts as a substrate to enhance stability. ECM–DPP6 interactions thus likely support filopodia formation and stability through binding to the RGD motif of the ECM to enhance cell adhesion. We performed an ECM binding assay to look for potential ECM protein partners for DPP6. Results presented in Fig. 8c,d show such an interaction of DPP6, specifically with fibronectin. We did not, however, find evidence for DPP6 interaction with collagen type 1, 4 or laminin. In this study, we identify a novel role for DPP6 in the regulation of dendritic filopodia formation and stability. Knockdown or genetic deletion of DPP6 resulted in fewer filopodia noted early in development. Moreover, live imaging experiments showed that the filopodia, in DPP6-lacking neurons, were unstable compared with those from WT neurons. These deficits could be rescued by exogenous expression of DPP6 and were not replicated in Kv4.2-KO neurons demonstrating a specific role for DPP6 in neuronal development independent of its role as a Kv4.2 auxiliary subunit in the hippocampal neurons. In the adult, DPP6-KO neurons showed fewer functional synapses and a sparser dendritic arbor. DPP6 appears to be acting postsynaptically, as decreased synaptic transmission was observed without affecting presynaptic properties. In addition, we provide evidence showing an interaction between DPP6 and Myosin-X, a molecular motor that functions in filopodia formation [32] . Finally, we showed that DPP6 interacts with the ECM protein fibronectin to enhance cell adhesion to the substratum. In total, these data present a structural role for DPP6 impacting dendritic morphology and synapse numbers beginning early in development and persisting into adulthood. The strong developmental role for DPP6 suggests a potential pathophysiological link to its genetic association with autism susceptibility [9] , highlighting the importance of further study into the role of DPP6 during normal circuit formation and synaptic development. Myosin-X is a plus-end-directed, high-duty-ratio myosin [32] , [33] that uses its motor activity to transport itself and its cargos to the tips of filopodia. Recent biochemical data demonstrate that Myosin-X can be converted from an inactive monomer to an active dimer [34] , which suggests that in cells, its ability to transport cargos to filopodia is regulated. Together with crystal structure data suggesting a conspicuously large extracellular domain for DPP6 [15] and previously reported ECM binding role for the related family member, DPP4/CD26 [19] , [20] , our results suggest a model where Myosin-X delivers DPP6 to the tips of filopodia where its extracellular domain interacts with fibronectin in the ECM to provide mechanical stability and aid in filopodial elongation, perhaps by preventing the retrograde flow of Myosin-10 and/or actin. The finding that DPP6 interacts with proteins in the ECM is also significant because it provides a function for its large extracellular domain. This domain of DPP6 (like that of DPP10 and other transmembrane DPPs) constitutes an overwhelming proportion of the protein. Yet, experiments with chimeric proteins lacking the extracellular domain of DPP6 (which was replaced by a series of Myc tags), showed that these mutants produce changes in expression and biophysical properties of Kv4 channels that were similar to those produced by the whole protein [8] . Here we found that the hippocampal neurons cultured from Kv4.2-KO mice do not show similar effects on filopodia formation and stability as reported here for those of DPP6-KO ( Fig. 5 ). Therefore, it appears that DPP6 has functions independent of its role as a Kv4 auxiliary subunit during development. These results support those showing that DPP6 does not require complex formation with Kv4 channels for intracellular trafficking, membrane expression and recycling [35] , [36] . In addition to impacting filopodia stability, loss of DPP6 had consequences for spine number and dendritic branching patterns in CA1 neurons in adult neurons. As no differences in branch numbers were found at DIV3, the sparser dendritic branching pattern in adulthood is likely a developmental effect. A sparse tree would be expected to produce a reduction in total spine number, but we also found that the remaining dendrites of adult DPP6-KO neurons exhibited decreased spine density compared with WT. This may too be the consequence of aberrant development in the absence of DPP6 or, perhaps, indicate that DPP6 functions in synapse stability throughout development and into adulthood. Interestingly, the loss of spine density in DPP6-KO dendrites was most prominent in distal dendrites, which corresponds to the effect of DPP6 on A-type K + current amplitudes; the loss was also most prominent in distal CA1 dendrites. Future studies will be necessary to determine if this indicates subcellular recognition and/or trans-synaptic signalling roles for DPP6 and, if so, whether or not DPP6 proteins functioning in this manner are also acting independent of Kv4 channels. Constructs DPP6-GFP or DPP6-mCherry constructs were prepared by PCR on construct rat pcDNA3-DPP6 (ref. 21 ) and subcloned into the pEGFP-N1 or pmCherry-N1 vector (Clontech, Mountain View, CA). Myosin-X-GFP constructs are previously described and characterized (Berg and Cheney [27] ). Additional details, including construction specifics and primer sequences, are given in the Supplementary Methods . Rat and mouse hippocampal neuron culture and transfection For details on the preparation of the primary hippocampal neuron cultures from E18-19 WT, DPP6-KO and Kv4.2-KO mice or Sprague–Dawley rats, please see Supplementary Methods . These methods were approved by NICHD’s Animal Care and Use Committee. Immunocytochemistry The cultured hippocampal neurons were fixed with freshly prepared 4% paraformaldehyde plus 4% sucrose in phosphate-buffered saline (PBS). Neurons were blocked with 10% normal goat serum in PBS and permeabilized with 0.2% Triton X-100 PBS for 10 min, immunostained with rabbit anti-MAP2 (1:1000, Chemicon), mouse anti-PSD-95 (1:200, NeuroMab), mouse anti-Synaptophysin (1:500, Millipore), mouse anti-Tau-1 (1:1000, Millipore) for 1 h at 37 °C, washed with PBS and incubated with Alexa Fluor 488 conjugated goat anti-rabbit (1:500, Invitrogen), Alexa Fluor 555 conjugated goat anti-mouse or Alexa Fluor 633 goat anti-rabbit for 1 h at 37 °C. Some neurons were counterstained with TRITC-phalloidin (1:500, Invitrogen) to visualize actin filaments. Cells were imaged with a Zeiss Axioplan 2 microscope or a Zeiss LSM510 confocal microscope (Carl Zeiss, Germany) using a 63 × objective with a 1.4 numerical aperture. Imaging and measurements are described in full in Supplementary Information . Time-lapse light microscopy To make time-lapse sequences, the WT or DPP6-KO P0 mouse [13] hippocampal neurons, in some cases expressing DPP6-GFP or GFP as a control, were cultured for 3–4 days on 25 mm round coverslips. Time series were acquired in differential interference contrast mode using 0.5% transmission of the 561 nm laser on the transmission path of a Zeiss Live Duo scan microscope. The neurons were maintained at 37 °C with 5% CO 2 in a humidified environment. The cells were exposed to light only during image acquisition (5–7 s per image). We used a × 63 per 1.40 Oil differential interference contrast M27 Plan-Apochromat objective. Time-lapse recordings of dendrites were carried out for 60 min during which time images were collected at a rate of one image every 30 s. Filopodia detected during the recording period and which remained for the duration were counted as new filopodia. All images were analysed using MetaMorph software. Staining and imaging analysis Six to eight-week-old male WT C57BL/6 and DPP6-KO mouse brain slices (250 μm thick) were prepared using a vibrating tissue slicer as described for the whole-cell electrophysiological recording methods listed below. Two milligrams of biocytin was added to 1 ml internal solution containing (in mM): 20 potassium chloride, 125 potassium gluconate, 10 HEPES (4-(2-hydroxyethyl)-1-piperazineethanesulfonic acid), 4 NaCl, 0.5 EGTA (ethylene glycol tetraacetic acid), 10 phosphocreatine, 4 ATP, 0.3 TrisGTP (pH 7.2 with NaOH) and was passively perfused into CA1 neurons. Somatic patches were maintained for 20 min to let biocytin diffuse throughout the neuron. Access (5~10 MΩ) was carefully monitored during all injections. After slowly withdrawing injection pipettes, slices were rapidly transferred to PBS containing 4% PFA. Tissue was fixed for 24 h before IHC staining. Biocytin-filled slices were single labelled with Alexa-488 conjugated streptavidin (1:500, Invitrogen) overnight at 4 °C after being permeabilized with 0.3% Triton X-100 in PBS. Following 4 × washes in PBS, slices were then cryoprotected using a 25% sucrose/PBS solution, and subsectioned into 70-μm thick slices using a freezing microtome, washed in PBS at 4 °C for 2–3 h and mounted on gelatin-coated slides using Mowiol mounting medium (Calbiochem, La Jolla, CA). Confocal image stacks of stained cells were performed at the NICHD Microscopy & Imaging Core facility using a Zeiss LSM 510 Inverted Meta with × 63 oil objective lens. Branching complexity was analysed by Sholl analysis [37] . Neurons were traced with the center of the soma as a focal point. Sholl measurements were obtained by quantifying the number of dendritic intersections crossing each 20-μm radius from soma. To calculate spine density, all dendrites located at a specific distance (40, 120, 240 μm from soma) were counted, and the number of spines along the length was counted to give a measure of spine per 20 μm length. Co-immunoprecipitation and western blotting To confirm an interaction between DPP6 and Myosin-X, we performed co-IP experiments either in native, detergent-solubilized mouse brain extracts or COS7 cells co-transfected with various DPP6 and Myosin-X constructs for 24–48 h. Mouse brain or cells were lysed in lysis buffer: 150 mM NaCl, 20 mM Tris-HCl, 1% NP40, 0.5% SDS and protease inhibitor mixture (Roche, Indianapolis, IN). Anti-DPP6 (2 μg per 500 μg protein, Abcam, Cambridge, MA), IgG (Invitrogen) as nonspecific control was then added to the lysate. The mixture was then incubated and rotated at 4 °C overnight. The antibody–antigen complex was immobilized by adsorption onto 50 μl of immobilized protein A (Pierce, Rockford, IL) and incubated for 2 h at room temperature. The protein-bead mixtures were washed 6 × with lysis buffer. The beads were resuspended in reducing SDS sample buffer and analysed on 3–8% Tris-acetate SDS polyacrylamide gels. The separated proteins were immunoblotted using DPP6 (1:2000) or Myosin-X antibody (1:4000, Cat# HPA024223, Sigma) and visualized by Alexa Fluor 680 secondary antibody (1:10,000, Invitrogen) and Alexa Fluor 800 secondary antibody (1:10,000, Rockland, Gilbertsville, PA). Immunoreactivity was detected with the Odyssey infrared imaging system (LI-COR Biosciences, Lincoln, Nebraska). Cell adhesion and ECM binding assay Adhesion of COS7 cells to a substratum was assayed as described [38] , [39] . Ninety-six-well plates coated with 0.1 mg ml −1 poly-L-lysine overnight at 4 °C were used for cell adhesion assay; ECM-coated 96-well plates (BD BioCoat, Bedford, MA) were used for binding assay. Plates were blocked with DPBS containing 2% BSA for 2 h. Transfected cells were harvested with enzyme-free cell dissociation buffer (Invitrogen), and then plated in DMEM with 1% BSA at a density of 60,000 cells per well. Cells were allowed to attach to the wells for 60 min at 37 °C, then non-adherent cells were washed away. The remaining adherent cells were fixed with 5% glutaraldehyde for 30 min and stained with 5 mg ml −1 crystal violet in 20% methanol for 30 min, washed with PBS and extracted with 0.2% Triton X-100 for 30 min. Microplates were colorimetrically evaluated at 576 nm. RGD or RAD treatment DIV3 mouse hippocampal neurons were treated with 250 μM RGD-containing peptide [Gly-Arg-Gly-Asp-Thr-Pro (GRGDTP)] (EMD Biosciences, San Diego, CA) or the control RAD-containing peptide [Gly-Arg-Ala-Asp-Ser-Pro (GRADSP)] (EMD Biosciences) for 1 h at 37 °C with 5% CO 2 , then neurons were fixed and immunostained with TRITC-phalloidin and density of filopodia quantified. Electrophysiology Six- to eight-week-old male C57BL/6 WT, Kv4.2-KO and DPP6-KO mice were anaesthetized by isoflurane prior to decapitation according to the methods approved by NICHD’s Animal Care and Use Committee. Acute brain slices (250-μm thick) were prepared using a vibrating tissue slicer as described previously [13] . The cultured hippocampal neurons were recorded on DIV 14–16. During recording, cultured neurons were bathed in extracellular solution containing (in mM) 145 NaCl, 3 KCl, 10 HEPES (4-(2-hydroxyethyl)-1-piperazineethanesulfonic acid), 8 dextrose, 2 CaCl 2 , 2 MgCl 2 . Somatic whole-cell recordings were performed at 32–33 °C for slices and 20 °C for cultured neurons, and were made from visually identified CA1 pyramidal neurons using differential interference contrast optics. Recording pipettes had tip resistances of 3–5 MΩ. Series resistance varied between 6 and 15 MΩ, and was carefully monitored throughout the experiments. No compensation for series resistance was employed. Neurons showed a resting membrane potential lower than −60 mV. Recordings in which the resting potential changed by more than ±5 mV of the initial value were excluded from the analysis. All electrophysiological data were recorded using a Multiclamp 700B amplifier. Signals were digitized at 10 kHz with a Digidata 1440 A and filtered at 2 kHz for miniature excitatory synaptic currents and at 4 kHz for PPF recordings. For recording miniature excitatory synaptic currents, recording pipettes were filled with intracellular solution containing (in mM) 100 Cs-gluconate, 5 MgCl 2 , 0.6 ethylene glycol tetraacetic acid, 8 NaCl, 40 HEPES (4-(2-hydroxyethyl)-1-piperazineethanesulfonic acid), 2 NaATP, 0.3 TrisGTP (pH 7.2 with KOH). TTX (1 μM), Bicuculline (20 μM) were included in the external solution during all mEPSC recordings. After whole-cell formation, a 5-min recovery period elapsed before data collection. Membrane potential was held at −65 mV. Each neuron was recorded continuously for 10 min. Synaptic currents were analysed with the Mini Analysis program (Synaptosoft Inc.). Only events showing a rise time and decay time less than 2 and 10 ms, respectively, and amplitude greater than 8 pA, were analysed. For PPF recordings, the patch electrode solution contained the same internal solution listed above for mEPSC recordings. Experiments were performed in 20 μM Bicuculline. A 50-ms interval elapsed between the 1st and 2nd stimulus pulse. Paired-pulse ratios are the ratio of the amplitude of the second EPSC to the first. All PPF recordings were analysed using Clampfit 10.1 and Microsoft Excel. Statistical significance was evaluated using Student’s t -test (unpaired, two tails). How to cite this article: Lin, L. et al. DPP6 regulation of dendritic morphogenesis impacts hippocampal synaptic development. Nat. Commun. 4:2270 doi: 10.1038/ncomms3270 (2013).